Blockade of IDO-kynurenine-AhR metabolic circuitry abrogates IFN-γ-induced immunologic dormancy of tumor-repopulating cells Interactions with the immune system may lead tumorigenic cells into dormancy. However, the underlying molecular mechanism is poorly understood. Using a 3D fibrin gel model, we show that IFN-γ induces tumour-repopulating cells (TRCs) to enter dormancy through an indolamine 2,3-dioxygenase 1 (IDO1)-kynurenine (Kyn)-aryl hydrocarbon receptor (AhR)-p27 dependent pathway. Mechanistically, IFN-γ signalling triggers differentiated tumour cell apoptosis via STAT1; however, when IDO1 and AhR are highly expressed as in TRCs, IFN-γ results in IDO1/AhR-dependent p27 induction that prevents STAT1 signalling, thus suppressing the process of cell death and activating the dormancy program. Blocking the IDO/AhR metabolic circuitry not only abrogates IFN-γ-induced dormancy but also results in enhanced repression of tumour growth by IFN-γ-induced apoptosis of TRCs both in vitro and in vivo . These data present a previously unrecognized mechanism of inducing TRC dormancy by IFN-γ, suggesting a potential effective cancer immunotherapeutic modality through the combination of IFN-γ and IDO/AhR inhibitors. Immunologic tumour dormancy, observed in clinical post-transplantation patients [1] , [2] , [3] , is a formidable barrier for further success of immunotherapies such as checkpoint inhibitor blockade [4] , oncolytic virus [5] and adoptive T-cell transfer [6] . Conceptually, immunologic tumour dormancy originates from the interaction between the immune system and tumour. However, to date, how the body’s immune responses induce the entry of tumour into dormancy remains elusive. Furthermore, immunologic tumour dormancy is also confounded by the inability to distinguish tumour mass dormancy from tumour cell dormancy. According to the 3E theory (elimination, equilibrium and escape) of cancer immunoediting proposed by Robert Schreiber and colleagues [7] , [8] , tumour mass dormancy represents the equilibrium of tumour growth and immune-mediated tumour killing, determining the outcome of tumour escape or elimination. On the other hand, tumour cell dormancy is defined at a cellular level as a process of immune factor-induced cell cycle arrest [9] . Recent studies showed that tumour cells in the equilibrium state are unedited and proliferate poorly; however, they can escape immune control and become edited and then grow into large tumour nests [10] , [11] , [12] . Therefore, such equilibrium state exemplifies cellular dormancy. Nevertheless, it is largely unknown why unedited highly immunogenic tumour cells in the dormant state are not recognized and destroyed by the adaptive immune system. Furthermore, under pressure from immunosurveillance, whether differentiation status affects the ability of tumour cells to undergo dormancy also remains unclear. Stem cell-like cancer cells that can repopulate tumours (TRC) [13] , [14] , [15] , [16] are a self-renewing, highly tumorigenic subpopulation of cancer cells and play crucial roles in the initiation, promotion and progression of tumorigenesis. Notably, certain properties of TRCs are now thought to be associated with tumour dormancy [17] , [18] , and even tumour dormancy and TRCs are thought as two sides of the same coin [19] . Like normal tissue stem cells, TRCs are characterized with self-renewal and differentiation potential but also possess the immunological properties to avoid immune-mediated destruction [20] , [21] . However, even though TRCs can escape the killing by cytotoxic immune cells such as CTLs and NK cells, it is possible that antitumour immune responses generate certain mechanisms to inhibit the growth of TRCs and render them dormant [12] , [22] , [23] . IFN-γ is a pleiotropic cytokine primarily produced by cytotoxic CTLs and NK cells and is known to function as a crucial antitumour immune factor. Upon binding to the type II IFN receptor, IFN-γ triggers the JAK/STAT signalling cascade that leads to the expression of a large array of interferon induced genes which can cause growth arrest, cell death or make tumour cells to upregulate MHC-I expression and antigen presentation, thus becoming more susceptible to MHC-restricted cytolytic killing [24] , [25] . However, IFN-γ can also upregulate immunosuppressive molecules such as PD-L1 and IDO, thereby facilitating tumour escape from immune elimination [26] . In addition to tumour elimination and tumour escape, IFN-γ has also been implicated in playing a role in tumour equilibrium where growth and expansion of tumorous cells are held in check by the immune system [23] , suggesting a possibility that IFN-γ is involved in cancer cell or even TRC dormancy. To date, whether and how IFN-γ participates in controlling cancer dormancy remains unknown. In this study, we provide evidence that IFN-γ induces the entry of TRCs into dormancy through the IDO-Kyn-AhR-p27 cascade. We also show TRC dormancy can be abrogated by inhibiting such key metabolic circuitry, thus allowing more effective tumour elimination. Linking tumour dormancy to stem-like tumour cells or TRCs would broaden the framework of the 3E theory of immunosurveillance and antitumour immunity, and provides a new direction to develop novel therapeutics and treatment strategies for preventing tumour recurrence and treatment resistance. IFN-γ induces murine TRC dormancy in vitro IFN-γ is known to be capable of inducing apoptosis or growth arrest of target tumour cells [27] , [28] , however, the mechanistic basis and physiological significance of these distinct antitumour outcomes has not been elucidated. We hypothesized that differentiation status of tumour cells might be a key determinant for IFN-γ-induced apoptosis or growth arrest. To test this hypothesis, we examined the response of differentiated tumour cells and stem-like TRCs to IFN-γ treatment. We have established a highly effective 3D fibrin gel culture system to generate TRCs [13] , [14] , [15] , [16] . Such fibrin gels correspond to 90 Pa in elastic stiffness and the TRCs were trapped individually in the 3D fibrin gels for colony formation. Such TRCs not only showed spheroid-like morphological changes resembling stem-like cells, but also as few as ten gel-selected cells were able to grow tumours in immunocompetent mice, confirming their stem-like properties in vivo [14] . By using this soft 3D fibrin gel method, we found that IFN-γ did not induce the death of B16 TRCs even at a high concentration; however, much lower dose of IFN-γ was enough to effectively kill control differentiated B16 cells cultured in rigid plastic plates ( Fig. 1a ), indicating that IFN-γ seems to be ineffective to stem-like TRCs. Surprisingly, even though IFN-γ didn’t induce apoptosis in B16 TRCs, their growth was markedly inhibited ( Fig. 1b ). Cell cycle analysis showed a G0/G1 arrest of these TRCs ( Fig. 1c ). Dormancy is an important physiological state during tumour development. Although the molecular nature has not been fully understood, tumour cell dormancy can be functionally defined as G0/G1 arrest, being neither apoptotic nor senescent, consuming less glucose, decreasing the reaction to stimulators as well as re-growing once inducers of dormancy are removed. In line with cell death resistance and cell cycle arrest of TRCs, we also found that IFN-γ treatment downregulated the expression of the PCNA gene, a cell proliferation marker and decreased glucose consumption by TRCs ( Fig. 1d,e ). In addition, compared to the positive control (IFN-γ+TNF-α), IFN-γ-treated TRCs did not undergo senesence as shown by β-galactosidase activity ( Fig. 1f ), suggesting that IFN-γ is capable of inducing dormancy of TRCs. Dormant tumour cells may decrease their response to xenobiotics, including chemotherapeutic drugs. Indeed, our data showed that dormant TRCs induced by IFN-γ were more resistant to methotrexate and paclitaxol ( Fig. 1g ). In addition to B16 melanoma, we found that IFN-γ could also induce TRCs from other types of murine tumour cells into dormancy ( Supplementary Fig. 1a ), representing a highly common phenomenon. Intriguingly, dormancy induction and maintenance appeared to involve different mechanisms. We found that TRC dormancy induced by high dose IFN-γ (200 ng ml −1 ) could be maintained by low dose (20 ng ml −1 ) ( Fig. 1h ). However, without pre-treatment of high dose, low doses of IFN-γ were unable to induce B16 TRCs into dormancy ( Supplementary Fig. 1b ). Collectively, these data suggest that IFN-γ is a key effector molecule of the immune system for TRC dormancy induction and maintenance in vitro . 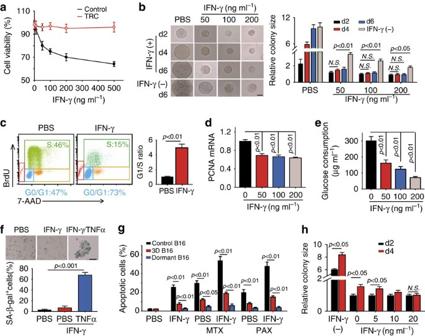Figure 1: IFN-γ induces TRC dormancyin vitro. (a) B16 cells in conventional rigid plate or B16 TRCs seeded in soft 3D fibrin gels were cultured for 3 days in the presence of different concentration of IFN-γ. Cell viability were analysed by flow cytometry. (b,c) B16 cells were seeded in soft 3D fibrin gels for 3 days, and then treated with different doses of IFN-γ for additional 2 days (d2), 4 days (d4) or 6 days (d6). For the bottom wells, IFN-γ was provided for the first 4 days and withdrawn for the last 2 days. Colony size was indicated (b), and cell cycle was analysed after 3 days IFN-γ treatment (100 ng ml−1) (c). The relative colony size was calculated by comparing the colony size in other groups with the colony size in the group of IFN-γ (50 ng ml−1) treated for 2 days, which was set to 1. Bar, 50 μm. (d,e) IFN-γ treatment decreased the expression of PCNA mRNA in B16 TRCs (d), and the glucose consumption (e). (f) B16 TRCs were treated with IFN-γ (100 ng ml−1) or IFN-γ/TNF-α (10 ng ml−1) for 72 h. SA-β gal staining was conducted. Bar, 50 μm. (g) control B16 cells from rigid plate, B16 TRCs, or dormant TRCs (72 h IFN-γ treatment) were treated with methotrexate (MTX, 250 ng ml−1) or paclitaxal (PAX, 2 μg ml−1) for 24 h. Cell viability was measured by flow cytometry. (h) TRC dormancy induced by high dose of IFN-γ was maintained by low dose of IFN-γ. B16 TRCs were treated with 200 ng ml−1IFN-γ for 2 days, then treated with different low doses of IFN-γ as indicated and cultured for another 2–4 days. The relative colony size was calculated by comparing the colony size in other groups with the colony size in the group of IFN-γ (0 ng ml−1) treated for 2 days, which was set to 1. Data shown are representative of three independent experiments and error bars represent mean±s.e.m., NS, no significant difference (Student’st-test). Figure 1: IFN-γ induces TRC dormancy in vitro . ( a ) B16 cells in conventional rigid plate or B16 TRCs seeded in soft 3D fibrin gels were cultured for 3 days in the presence of different concentration of IFN-γ. Cell viability were analysed by flow cytometry. ( b , c ) B16 cells were seeded in soft 3D fibrin gels for 3 days, and then treated with different doses of IFN-γ for additional 2 days (d2), 4 days (d4) or 6 days (d6). For the bottom wells, IFN-γ was provided for the first 4 days and withdrawn for the last 2 days. Colony size was indicated ( b ), and cell cycle was analysed after 3 days IFN-γ treatment (100 ng ml −1 ) ( c ). The relative colony size was calculated by comparing the colony size in other groups with the colony size in the group of IFN-γ (50 ng ml −1 ) treated for 2 days, which was set to 1. Bar, 50 μm. ( d , e ) IFN-γ treatment decreased the expression of PCNA mRNA in B16 TRCs ( d ), and the glucose consumption ( e ). ( f ) B16 TRCs were treated with IFN-γ (100 ng ml −1 ) or IFN-γ/TNF-α (10 ng ml −1 ) for 72 h. SA-β gal staining was conducted. Bar, 50 μm. ( g ) control B16 cells from rigid plate, B16 TRCs, or dormant TRCs (72 h IFN-γ treatment) were treated with methotrexate (MTX, 250 ng ml −1 ) or paclitaxal (PAX, 2 μg ml −1 ) for 24 h. Cell viability was measured by flow cytometry. ( h ) TRC dormancy induced by high dose of IFN-γ was maintained by low dose of IFN-γ. B16 TRCs were treated with 200 ng ml −1 IFN-γ for 2 days, then treated with different low doses of IFN-γ as indicated and cultured for another 2–4 days. The relative colony size was calculated by comparing the colony size in other groups with the colony size in the group of IFN-γ (0 ng ml −1 ) treated for 2 days, which was set to 1. Data shown are representative of three independent experiments and error bars represent mean±s.e.m., NS, no significant difference (Student’s t -test). Full size image IFN-γ induces murine TRC dormancy in vivo To establish the physiological significance, we next examined whether IFN-γ could induce TRC dormancy in vivo . To this end, C57BL/6 mice bearing subcutaneously implanted B16 melanomas with 5 × 5 mm in size were intratumorally treated with PBS or IFN-γ (10 μg per day) for 3 days and then tumour cells were isolated. Cell cycle analysis showed that IFN-γ treatment increased the G0/G1 proportion in the living tumour cells from 7.6 to 64.4% ( Fig. 2a ). CD133 is commonly used to mark stem cell-like cancer cells, including melanoma cells [29] , [30] . We sorted CD133 + tumour cells from B16 melanoma to perform cell cycle analysis and found that IFN-γ treatment induces most of them into dormancy ( Fig. 2b ). β-galactosidase staining showed that the tumour cells did not enter senesence ( Fig. 2c ), suggesting that B16 TRCs may be induced to enter dormancy by IFN-γ. In addition to B16 melanoma, a murine malignant ascites model was also tested by intraperitoneal injection of H22 hepatocellular carcinoma cells into BALB/c mice [31] . Twenty four hours later, these mice were treated with IFN-γ. Consequently, dormant H22 TRCs in the abdominal cavity markedly increased from 18.5 to 66.0% ( Supplementary Fig. 1c ). In a different setting, C57BL/6 mice were injected s.c. with 5 × 10 3 B16 TRCs for 3 days and then treated with IFN-γ (10 μg every 2 days). On day 5, a tiny melanoma nest at the injection site was confirmed by immunohistochemical and H&E stainings. On day 20, melanoma in the PBS control group had grown to be 5 × 5 mm, while IFN-γ treatment kept the original tumour size as observed on day 5, further suggesting that IFN-γ induces TRC dormancy in vivo ( Fig. 2d ). More convincingly, the administration of IFN-γ neutralizing antibody beginning at day 10 resulted in the regrowth of the tumour in mice, confirming the dormancy induced by IFN-γ is reversible ( Fig. 2e ). To explore the potential clinical significance of this in vivo immunological dormancy, we adoptively transferred OVA-specific T cells to mice with OVA-B16 melanoma for twice. We found that the unkilled OVA-B16 cells appeared to enter dormancy by cell cycle arrest and with negative β-gal staining ( Fig. 2f,g ). In addition, flow cytometric analysis also showed that the CD133 + OVA-B16 cells entered G0/G1 cell cycle arrest ( Supplementary Fig. 1d ). Intriguingly, using antibody to neutralize IFN-γ in the mice prevented the above CTL-mediated tumour cell dormancy, suggesting that tumour-specific CTLs might release IFN-γ to induce unkilled TRCs into dormancy. Taken together, the data demonstrated that IFN-γ can induce functional tumour dormancy in vivo with potential clinical significance. 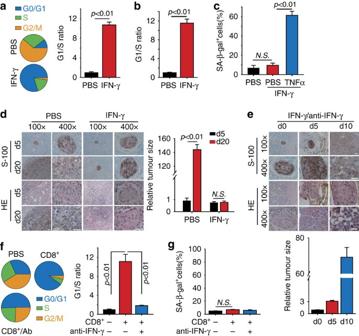Figure 2: IFN-γ induces TRC dormancyin vivo. (a,b) C57BL/6 mice with 5 × 5 mm B16 melanoma were intratumorally treated with 10 μg IFN-γ once per day for 3 days (n=6 per group). Isolated primary tumour cells were assayed for cell cycle analysis (a). Or CD133hightumour cells were sorted from tumour by FACS and performed cell cycle analysis (b). (c) the same asa, but mice were treated with 10 μg IFN-γ in the presence or absence of TNF-α once per day for 3 days. Isolated primary tumour cells were stained with SA-β gal. (d) B16 TRCs (5 × 103) were subcutaneously injected to mice. On day 3, 10 μg IFN-γ was directly injected into tumour site once every 2 days (n=8 per group). On day 5 and day 20, tumour cell-injected tissues were analysed by immunostaining against S100β or H&E staining. The tumour size was presented photographically (left) and graphically (right). Bar, 25 μm. (e) 5 × 103B16 TRCs were subcutaneously injected to C57BL/6 mice, and then mice were intratumorally treated with IFN-γ (10 μg per day) for 10 days, and then further treated with IFN-γ or IFN-γ+anti-IFN-γ antibody (250 μg per day) once every two days (n=8 per group). Tissues at the injection site were collected on day 10 (d0), day 15 (d5) or day 20 (d10), and used for immunostaining against S100β or H&E staining. Bar, 25 μm. (f,g) Mice were s.c. injected with 2 × 105OVA-B16 TRCs (n=8 per group). When the tumour size reached 3 × 3 mm, mice were adoptively transferred with OVA-specific CD8+T cells (1 × 107cells per mouse) once per two days for twice. Some mice were pretreated with anti-IFN-γ antibody (250 μg per day) once per two days for twice. The isolated primary tumour cells were performed cell cycle analysis (f) and SA-β gal staining (g). In this figure, the data represented mean±s.e.m., NS, no significant difference (Student’st-test). Figure 2: IFN-γ induces TRC dormancy in vivo . ( a , b ) C57BL/6 mice with 5 × 5 mm B16 melanoma were intratumorally treated with 10 μg IFN-γ once per day for 3 days ( n =6 per group). Isolated primary tumour cells were assayed for cell cycle analysis ( a ). Or CD133 high tumour cells were sorted from tumour by FACS and performed cell cycle analysis ( b ). ( c ) the same as a , but mice were treated with 10 μg IFN-γ in the presence or absence of TNF-α once per day for 3 days. Isolated primary tumour cells were stained with SA-β gal. ( d ) B16 TRCs (5 × 10 3 ) were subcutaneously injected to mice. On day 3, 10 μg IFN-γ was directly injected into tumour site once every 2 days ( n =8 per group). On day 5 and day 20, tumour cell-injected tissues were analysed by immunostaining against S100β or H&E staining. The tumour size was presented photographically (left) and graphically (right). Bar, 25 μm. ( e ) 5 × 10 3 B16 TRCs were subcutaneously injected to C57BL/6 mice, and then mice were intratumorally treated with IFN-γ (10 μg per day) for 10 days, and then further treated with IFN-γ or IFN-γ+anti-IFN-γ antibody (250 μg per day) once every two days ( n =8 per group). Tissues at the injection site were collected on day 10 (d0), day 15 (d5) or day 20 (d10), and used for immunostaining against S100β or H&E staining. Bar, 25 μm. ( f , g ) Mice were s.c. injected with 2 × 10 5 OVA-B16 TRCs ( n =8 per group). When the tumour size reached 3 × 3 mm, mice were adoptively transferred with OVA-specific CD8 + T cells (1 × 10 7 cells per mouse) once per two days for twice. Some mice were pretreated with anti-IFN-γ antibody (250 μg per day) once per two days for twice. The isolated primary tumour cells were performed cell cycle analysis ( f ) and SA-β gal staining ( g ). In this figure, the data represented mean±s.e.m., NS, no significant difference (Student’s t -test). Full size image IDO-Kyn-AhR-p27 cascade mediates murine TRC dormancy Next, we explored how IFN-γ induced TRCs into dormancy. Indoleamine-2,3-dioxygenase 1 (IDO1), an enzyme which catalyses tryptophan metabolism, is known to be upregulated by IFN-γ [32] , [33] . As an essential amino acid, trptophan degradation by IDO1 might negatively influence protein synthesis and cell growth, leading to TRC dormancy. Consistent with this possibility, IDO1 overexpression by tranfecting IDO1-expressing plasmid resulted in G0/G1 arrest and TRC dormancy ( Fig. 3a,b ). In further support of this finding, we found that dormancy could be reversed by siRNA knockdown of IDO1 ( Fig. 3c and Supplementary Fig. 2a ). Kyn is a major metabolic intermediate of IDO1-catalysed tryptophan. Intriguingly, the addition of Kyn to the fibrin gels inhibited the growth of B16 TRCs, which was reversed by the removal of Kyn ( Fig. 3d,e ). Besides Kyn, other tryptophan metabolites such as kynurenic acid (KYNA) and indoxyl sulfate also act as endogenous ligands to activate AhR [34] , [35] . However, we found that neither KYNA nor indoxyle sulfate could inhibit the growth of B16 TRCs, even at high concentrations ( Supplementary Fig. 2b,c ). Likewise, melatonin as a tryptophan metabolite also did not induce TRCs into dormancy ( Supplementary Fig. 2d ), suggesting that TRC dormancy may be induced through the IDO-Kyn pathway. Additionally, we excluded the above TRC dormancy as a result of tryptophan consumption, which can cause the phosphorylation of eIF2α, dependent on GCN2, and consequently cause arrest in protein synthesis [36] . This is based on results showing that IFN-γ also induced dormancy in GCN2-knockdown B16 TRCs ( Supplementary Fig. 2e ). In addition, IFN-γ can also upregulate the expression of PD-L1 and iNOS in tumour cells and immune cells [37] , [38] . Intriguingly, we found that IFN-γ effectively stimulated the upregulation of PD-L1 in differentiated B16 cells, but not in B16 TRCs ( Supplementary Fig. 2f ). Also the expression of iNOS in TRCs seemed not to be regulated by IFN-γ ( Supplementary Fig. 2f ). Moreover, the knockdown of either PD-L1 or iNOS did not affect IFN-γ-induced B16 TRC dormancy ( Supplementary Fig. 2g ), suggesting that IFN-γ selectively mobilizes the IDO1 pathway to mediate TRC dormancy. 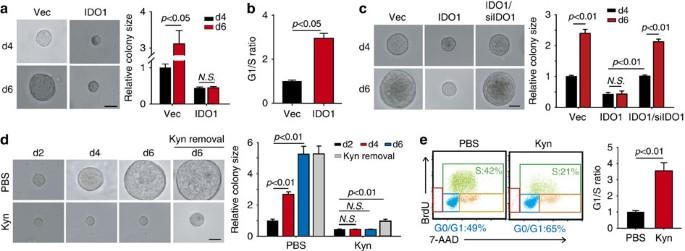Figure 3: IDO-Kyn metabolic circuitry mediates TRC dormancy. (a,b) IDO1-overexpressing B16 cells were seeded in soft 3D fibrin gels for 4 days (d4) or 6 days (d6). The colony size was indicated (a) and the cell cycle was analysed (b). The relative colony size was calculated by comparing the colony size in other groups with the colony size in the Vec (d4) group, which was set to 1. Bar, 50 μm. (c) IDO1- B16 cells were transfected with IDO1 siRNA or scramble siRNA and then seeded in soft 3D fibrin gels and cultured for the indicated days. The colony size is presented photographically and graphically. The relative colony size was calculated by comparing the colony size in groups with that in the Vec (d4) group, which was set to 1. Bar, 50 μm. (d) Kyn inhibited B16-TRC growth. B16-TRCs cultured in 3D soft gels for 2 days were treated with 150 μM Kyn for 2–4 days and at day 5, Kyn was removed from the supernatant and continued to culture for another 2 days. The relative colony size was calculated by comparing the colony size in other groups with the colony size in the PBS (d2) group, which was set to 1. Bar, 50 μm. (e) The same asd, but the TRCs were collected 72 h after Kyn treatment and performed cell cycle analysis. Data shown are representative of three independent experiments and error bars represent mean±s.e.m., NS, no significant difference (Student’st-test). Figure 3: IDO-Kyn metabolic circuitry mediates TRC dormancy. ( a , b ) IDO1-overexpressing B16 cells were seeded in soft 3D fibrin gels for 4 days (d4) or 6 days (d6). The colony size was indicated ( a ) and the cell cycle was analysed ( b ). The relative colony size was calculated by comparing the colony size in other groups with the colony size in the Vec (d4) group, which was set to 1. Bar, 50 μm. ( c ) IDO1- B16 cells were transfected with IDO1 siRNA or scramble siRNA and then seeded in soft 3D fibrin gels and cultured for the indicated days. The colony size is presented photographically and graphically. The relative colony size was calculated by comparing the colony size in groups with that in the Vec (d4) group, which was set to 1. Bar, 50 μm. ( d ) Kyn inhibited B16-TRC growth. B16-TRCs cultured in 3D soft gels for 2 days were treated with 150 μM Kyn for 2–4 days and at day 5, Kyn was removed from the supernatant and continued to culture for another 2 days. The relative colony size was calculated by comparing the colony size in other groups with the colony size in the PBS (d2) group, which was set to 1. Bar, 50 μm. ( e ) The same as d , but the TRCs were collected 72 h after Kyn treatment and performed cell cycle analysis. Data shown are representative of three independent experiments and error bars represent mean±s.e.m., NS, no significant difference (Student’s t -test). Full size image Aryl hydrocarbon receptor (AhR) plays an essential role in regulation of gene expression in a wide variety of cells. As a cytoplasmic transcription factor, AhR can be activated by exogenous xenobiotics such as 2,3,7,8-tetrachlorodibenzo-p-dioxin [39] or by endogenous metabolites including Kyn [40] . Here, we found that the addition of Kyn to B16 TRCs resulted in the translocation of AhR to the nucleus, demonstrated by fluorescent microscopy and western blot ( Fig. 4a,b ). As nuclear localization reflects an active form of AhR, this result suggested that AhR signalling might be involved in the induction of TRC dormancy. In support of this idea, AhR knockdown indeed blocked the dormancy induced by either IDO1 overexpression or Kyn ( Fig. 4c,d and Supplementary Fig. 3a,b ). Collectively, these data suggest that TRC dormancy might be mediated via an IDO-Kyn-AhR pathway. 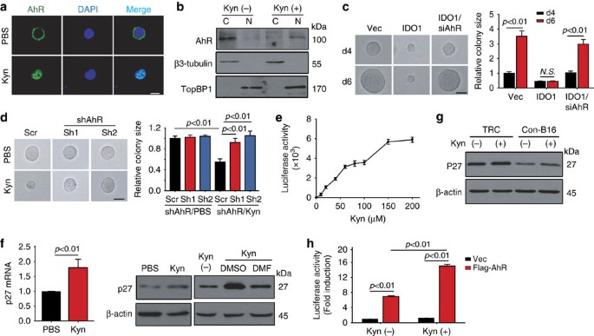Figure 4: TRC dormancy is regulated by Kyn-AhR-p27 pathway. (a) Kyn promoted the translocation of AhR from the cytosol to nucleus by immunostaining assay. Bar, 10 μm. (b) Cell fraction of cytosol (C) and nucleus (N) was analysed by western blot. (c) Stably IDO1-B16 cells were transfected with scramble or AhR siRNA and seeded in 3D soft fibrin gels and cultured for the indicated days. The colony size is presented photographically and graphically. The relative colony size was calculated by comparing the colony size in groups with that in the Vec (d4) group, which was set to 1. Bar, 50 μm. (d) B16 cells were stably transfected with scramble shRNA, AhR shRNA1 or AhR shRNA2, and cultured in soft 3D fibrin gels with or without Kyn (150 μM) for 48 h. Scramble-B16 TRCs were used as control. The colony size is presented photographically and graphically after Kyn treatment for 48 h. The relative colony size was calculated by comparing the colony size in groups with that in the ShAhR/PBS group, which was set to 1. Bar, 50 μm. (e) B16 TRCs were treated with different concentration of Kyn. AhR activity was determined by luciferase assay. (f) B16-TRCs were treated with Kyn (150 μM) in the presence or absence of DMF (20 μM). The expression of p27 was determined by real-time PCR (left) and western blot (right). (g) the expression of p27 in TRCs or control B16 cells with or without IFN-γ treatment. (h) Kyn enhanced the luciferase activity of p27 promoter. B16-TRCs were transiently transfected with a luciferase reporter plasmid of pGL3/p27 promoter with or without Flag-AhR in the presence or absence of Kyn for 24 h. Data shown are representative of three independent experiments and error bars represent mean±s.e.m. (Student’st-test). Figure 4: TRC dormancy is regulated by Kyn-AhR-p27 pathway. ( a ) Kyn promoted the translocation of AhR from the cytosol to nucleus by immunostaining assay. Bar, 10 μm. ( b ) Cell fraction of cytosol (C) and nucleus (N) was analysed by western blot. ( c ) Stably IDO1-B16 cells were transfected with scramble or AhR siRNA and seeded in 3D soft fibrin gels and cultured for the indicated days. The colony size is presented photographically and graphically. The relative colony size was calculated by comparing the colony size in groups with that in the Vec (d4) group, which was set to 1. Bar, 50 μm. ( d ) B16 cells were stably transfected with scramble shRNA, AhR shRNA1 or AhR shRNA2, and cultured in soft 3D fibrin gels with or without Kyn (150 μM) for 48 h. Scramble-B16 TRCs were used as control. The colony size is presented photographically and graphically after Kyn treatment for 48 h. The relative colony size was calculated by comparing the colony size in groups with that in the ShAhR/PBS group, which was set to 1. Bar, 50 μm. ( e ) B16 TRCs were treated with different concentration of Kyn. AhR activity was determined by luciferase assay. ( f ) B16-TRCs were treated with Kyn (150 μM) in the presence or absence of DMF (20 μM). The expression of p27 was determined by real-time PCR (left) and western blot (right). ( g ) the expression of p27 in TRCs or control B16 cells with or without IFN-γ treatment. ( h ) Kyn enhanced the luciferase activity of p27 promoter. B16-TRCs were transiently transfected with a luciferase reporter plasmid of pGL3/p27 promoter with or without Flag-AhR in the presence or absence of Kyn for 24 h. Data shown are representative of three independent experiments and error bars represent mean±s.e.m. (Student’s t -test). Full size image Once inside the nucleus, AhR begins to function as a transcription factor by binding to the specific DNA sequence region called dioxin-responsive element (DRE) to activate target gene expression [41] . By performing a DRE-luciferase assay, we demonstrated a Kyn dose dependent activation of the DRE-luciferase reporter ( Fig. 4e ), suggesting that AhR indeed operates directly downstream of Kyn in TRCs. To link AhR activation to TRC dormancy induction, we postulated that Kyn-AhR might upregulate the expression of cell cycle inhibitor(s) in TRCs. Therefore, a panel of cell cycle-regulatory molecules including cyclin D1, cyclin D3, cyclin A2, cyclin E, CDK2, p18, p21, p27 and p53 were screened and p27 was identified ( Supplementary Fig. 3c,d ). Firstly, Kyn treatment upregulated p27 expression at both mRNA and protein levels in TRCs, which could be blocked by an AhR inhibitor ( Fig. 4f ). Secondly, when dormant TRCs were seeded back to rigid plastic plate to induce their differentiation, p27 expression was remarkably decreased even in the presence of Kyn ( Fig. 4g ). Thirdly, co-transfection of p27 promoter luciferase reporter (pGL3/p27) and Flag-AhR vector resulted in a 14-fold increase of the luciferase activity in the presence of Kyn ( Fig. 4h ). Taken together, these data suggest that TRC dormancy is mediated by an IDO-Kyn-AhR-p27 pathway. IDO-Kyn-AhR crosstalks with STAT1 signalling via p27 Next, we investigated the effect of IFN-γ on IDO-Kyn-AhR cascade in TRCs. Interestingly, we found that the baseline expression of IDO1 was significantly higher in B16 TRCs relative to the control of differentiated B16 cells cultured on rigid plastic, and further upregulated by IFN-γ ( Fig. 5a and Supplementary Fig. 4a ). In line with IDO1 upregulation, Kyn levels were also increased upon IFN-γ stimulation ( Supplementary Fig. 4b ). Moreover, AhR was consistently higher in B16 TRCs and further upregulated by IFN-γ stimulation ( Fig. 5b ). Like Kyn, the addition of IFN-γ also promoted the translocation of AhR to the nucleus of TRCs ( Fig. 5c,d ), as well as the upregulation of p27 expression in TRCs, which could be blocked by 3′,4′-Dimethoxyflavone (DMF), an AhR inhibitor ( Fig. 5e and Supplementary Fig. 4c ). Together, these data suggest that IFN-γ activates IDO-Kyn-AhR cascade of TRCs. 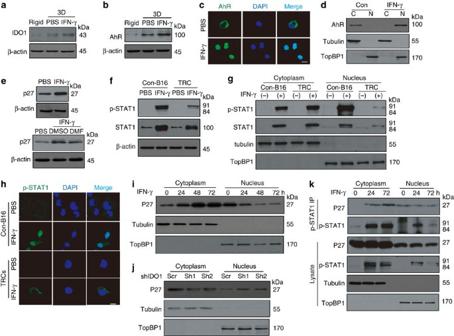Figure 5: IFN-γ activated IDO-Kyn-AhR cascade crosstalks with STAT1 pathway via p27. (a) the expression of IDO1 in control B16 cells, B16 TRCs or IFN-γ-treated B16 TRCs was determined by western blot. (b) the expression of AhR in control B16 cells, B16 TRCs or IFN-γ-treated B16 TRCs was determined by western blot. (c,d) B16 TRCs were treated with 100 ng ml−1IFN-γ for 3 days. The nuclear localization of AhR was determined by immuno-fluorescence staining (c) and western blot (d). Cytoplasmic β3-tubulin and nuclear TopBp1 were used as controls. (e) B16 TRCs were treated with IFN-γ (100 ng ml−1) or IFN-γ+DMF (20 μM) for 3 days. The expression of p27 was determined by western blot. (f–h) B16 TRCs were treated with or without IFN-γ (100 ng ml−1) for 3 days. Phosphorylated STAT1 in whole cell lysate (f) or cytoplasmic and nuclear fractions (g) was analysed by western blot. Immunostaining of p-STAT1 (green) and DAPI (blue) was represented (h). Bar, 10 μm. (i) B16 TRCs were treated with IFN-γ (100 ng ml−1) for indicated time. Cytoplasmic and nuclear p27 was analysed by western blot. (j) B16 TRCs, stably transfected with scramble shRNA or IDO1 shRNAs, were treated with IFN-γ (100 ng ml−1) for 72 h. Cytoplasmic and nuclear expression of p27 was analysed by western blot. (k) B16-TRCs were treated with IFN-γ (100 ng ml−1) for 24 or 72 h and the cytoplasmic and nuclear fractions were collected. Anti-phospho-STAT1 immunoprecipitates from both cytoplasm and nucleus were immunoblotted with anti-p27 and anti-phospho-STAT1 antibodies. Images shown are representative of three independent experiments. Figure 5: IFN-γ activated IDO-Kyn-AhR cascade crosstalks with STAT1 pathway via p27. ( a ) the expression of IDO1 in control B16 cells, B16 TRCs or IFN-γ-treated B16 TRCs was determined by western blot. ( b ) the expression of AhR in control B16 cells, B16 TRCs or IFN-γ-treated B16 TRCs was determined by western blot. ( c , d ) B16 TRCs were treated with 100 ng ml −1 IFN-γ for 3 days. The nuclear localization of AhR was determined by immuno-fluorescence staining ( c ) and western blot ( d ). Cytoplasmic β3-tubulin and nuclear TopBp1 were used as controls. ( e ) B16 TRCs were treated with IFN-γ (100 ng ml −1 ) or IFN-γ+DMF (20 μM) for 3 days. The expression of p27 was determined by western blot. ( f – h ) B16 TRCs were treated with or without IFN-γ (100 ng ml −1 ) for 3 days. Phosphorylated STAT1 in whole cell lysate ( f ) or cytoplasmic and nuclear fractions ( g ) was analysed by western blot. Immunostaining of p-STAT1 (green) and DAPI (blue) was represented ( h ). Bar, 10 μm. ( i ) B16 TRCs were treated with IFN-γ (100 ng ml −1 ) for indicated time. Cytoplasmic and nuclear p27 was analysed by western blot. ( j ) B16 TRCs, stably transfected with scramble shRNA or IDO1 shRNAs, were treated with IFN-γ (100 ng ml −1 ) for 72 h. Cytoplasmic and nuclear expression of p27 was analysed by western blot. ( k ) B16-TRCs were treated with IFN-γ (100 ng ml −1 ) for 24 or 72 h and the cytoplasmic and nuclear fractions were collected. Anti-phospho-STAT1 immunoprecipitates from both cytoplasm and nucleus were immunoblotted with anti-p27 and anti-phospho-STAT1 antibodies. Images shown are representative of three independent experiments. Full size image JAK-STAT1 is the key downstream pathway to mediate IFN-γ signalling [24] . Although STAT1 phosphorylation was induced by IFN-γ in both TRCs and differentiated B16 cells, reduced phosphorylation was observed in TRCs ( Fig. 5f ). Surprisingly, in contrast to control B16 cells, upon IFN-γ stimulation for 72 h, p-STAT1 was mainly located in the cytosol of TRCs rather than in the nucleus ( Fig. 5g,h ). Moreover, the time course study showed that p-STAT1 could enter the nucleus of control B16 cells and TRCs after 24-h IFN-γ treatment, while 72-h later, nuclear p-STAT1 was mainly found in control B16 cells but not B16 TRCs ( Supplementary Fig. 4d,e ). To understand the mechanism of blocking the entry of p-STAT1 into the nucleus of TRCs, we wondered whether p27 was involved in the process, considering the activation of IDO-Kyn-AhR-p27 by IFN-γ. In favour of this concept, we found that upon IFN-γ stimulation, a cytoplasmic increase, but nuclear decrease of p27 in TRCs was observed in a time-dependent manner ( Fig. 5i ), which was reversed by knockdown of IDO1 or AhR ( Fig. 5j and Supplementary Fig. 4f,g ). A co-immunoprecipitation assay further showed that p-STAT1 and p27 were co-localized in the cytosol of IFN-γ-treated TRCs ( Fig. 5k ). Taken together, these data suggest that IFN-γ simultaneously activates JAK-STAT1 and IDO-Kyn-AhR-p27 signallings, and we propose that p27 binding might prevent the translocation of p-STAT1 from the cytosol to the nucleus. Blocking IDO-Kyn-AhR disrupts TRC dormancy in vitro Subsequently, we wondered whether switching IFN-γ-mediated IDO1-Kyn-AhR cascade to STAT1 signalling influenced dormant TRCs. We found when IFN-γ and AhR inhibitor DMF were added to B16 TRC fibrin gels, both TRC colony size and number were decreased in a dose-dependent manner ( Fig. 6a,b ). Consistently, a similar result was also obtained from AhR-knockdown TRCs ( Supplementary Fig. 5a,b ). In addition to AhR, our data showed that IDO1 inhibitor 1-MT or IDO1 shRNAs also reduced B16 TRC colony number and size in the presence of IFN-γ ( Fig. 6c,d and Supplementary Fig. 5c,d ). B16 TRC apoptosis by 1-MT or DMF was also observed in the presence of IFN-γ ( Supplementary Fig. 5e ). Thus, switching the mode of STAT1 signalling by blocking IDO-Kyn-AhR cascade could disrupt IFN-γ-induced TRC dormancy. Translocation of p-STAT1 into the nucleus may trigger IFN-γ-induced cell death by activating caspases 3 and 7 (refs 42 , 43 ). In line with this notion, cleaved caspases 3 and 7 were found to be present at high levels in differentiated B16 cells upon IFN-γ stimulation, which on the other hand were present at low levels in TRCs ( Fig. 6e ). However, blockade of IDO-Kyn-AhR cascade by 1-MT or DMF led to an increase of cleaved (active) caspases 3 and 7 in TRCs ( Fig. 6f ), paralleled with increased translocation of p-STAT1 in the nucleus, as shown by immunofluorescent staining ( Fig. 6g ). Increased active caspases 3 and 7 were also observed from IDO1- or AhR-knockdown TRCs by western blot ( Supplementary Fig. 5f ). We thus prepared cytosolic and nuclear lysates of TRCs, and further confirmed that IDO1 or AhR knockdown caused increased translocation of p-STAT1 into the nucleus upon IFN-γ stimulation ( Supplementary Fig. 5g ). Consistent with IDO1 or AhR knockdown, p27 knockdown also promoted translocation of p-STAT1 into the nucleus of TRCs ( Supplementary Fig. 5h ), and subsequent cell death ( Supplementary Fig. 5i,j ). To further confirm this finding from a different angle, we used fludarabine, a STAT1 inhibitor, or STAT1 shRNA to block STAT1 activity to directly examine the role of STAT1 in apoptotic induction of TRCs by IFN-γ stimulation. In this case, 1-MT or DMF did not cause the cell death of TRCs, but rather relieved IFN-γ-induced TRC dormancy and allowed TRC proliferation ( Supplementary Fig. 6a–c ). Together, these data suggest that blocking the IDO-Kyn-AhR cascade may disrupt IFN-γ-induced TRC dormancy. 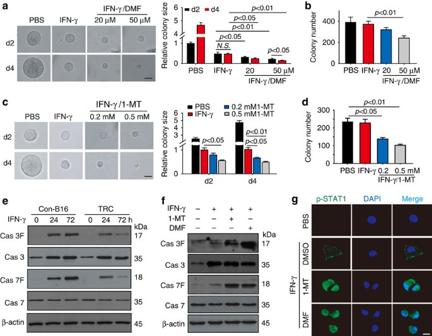Figure 6: Switching IFN-γ-mediated IDO-Kyn-AhR cascade to STAT1 signalling targets TRC dormancy. (a,b) B16 cells (1.25 × 103) were seeded in soft 3D fibrin gels. Two days later, IFN-γ was added for further 2 days (d2) or 4 days (d4) culture in the presence or absence of different concentration of DMF. The colony size was presented (a) and colony number was counted (b). The relative colony size was calculated by comparing the colony size in other groups with the colony size in the PBS (d2) group, which was set to 1. The data represent mean±s.e.m. (n=3). Bar, 50 μm. (c,d) The above B16 TRCs were cultured in the presence or absence of different concentration of 1-MT. The colony size was presented (c) and colony number was counted (d). The relative colony size was calculated by comparing the colony size in other groups with the colony size in the PBS (d2) group, which was set to 1. The data represent mean±s.e.m. (n=3). Bar, 50 μm. (e) control B16 cells or B16 TRCs were treated with 100 ng ml−1IFN-γ for 24 or 72 h (n=3). Caspase 3 (Cas 3), caspase 7 (Cas 7) and their cleaved forms (Cas 3F and Cas 7F) were determined by western blot. (f) B16-TRCs were treated with IFN-γ (100 ng ml−1) plus 1-MT (0.2 mM) or DMF (20 μM) for 72 h (n=3). Caspases were analysed by western blot. (g) B16-TRCs were treated with IFN-γ (100 ng ml−1), IFN-γ/1-MT (0.2 mM) or IFN-γ/DMF (20 μM) for 72 h. Immunostaining of p-STAT1 (green) and DAPI (blue) was shown as the representative of three independent experiments. Bar, 10 μm. Figure 6: Switching IFN-γ-mediated IDO-Kyn-AhR cascade to STAT1 signalling targets TRC dormancy. ( a , b ) B16 cells (1.25 × 10 3 ) were seeded in soft 3D fibrin gels. Two days later, IFN-γ was added for further 2 days (d2) or 4 days (d4) culture in the presence or absence of different concentration of DMF. The colony size was presented ( a ) and colony number was counted ( b ). The relative colony size was calculated by comparing the colony size in other groups with the colony size in the PBS (d2) group, which was set to 1. The data represent mean±s.e.m. ( n =3). Bar, 50 μm. ( c , d ) The above B16 TRCs were cultured in the presence or absence of different concentration of 1-MT. The colony size was presented ( c ) and colony number was counted ( d ). The relative colony size was calculated by comparing the colony size in other groups with the colony size in the PBS (d2) group, which was set to 1. The data represent mean±s.e.m. ( n =3). Bar, 50 μm. ( e ) control B16 cells or B16 TRCs were treated with 100 ng ml −1 IFN-γ for 24 or 72 h ( n =3). Caspase 3 (Cas 3), caspase 7 (Cas 7) and their cleaved forms (Cas 3F and Cas 7F) were determined by western blot. ( f ) B16-TRCs were treated with IFN-γ (100 ng ml −1 ) plus 1-MT (0.2 mM) or DMF (20 μM) for 72 h ( n =3). Caspases were analysed by western blot. ( g ) B16-TRCs were treated with IFN-γ (100 ng ml −1 ), IFN-γ/1-MT (0.2 mM) or IFN-γ/DMF (20 μM) for 72 h. Immunostaining of p-STAT1 (green) and DAPI (blue) was shown as the representative of three independent experiments. Bar, 10 μm. Full size image Disruption of murine TRC dormancy in vivo Next, we investigated whether switching IDO-Kyn-AhR cascade to the STAT1 pathway could abrogate dormant TRCs in vivo . In this regard, B16 TRC tumour-bearing mice (5 × 5 mm in size) were intratumorally treated with 10 μg IFN-γ once daily for 3 days. It was found that IFN-γ treatment significantly increased both IDO1 and p27 expression and caused AhR translocation from the cytoplasm to the nucleus ( Fig. 7a ). Consistent with the B16 melanoma model, IFN-γ treatment also upregulated IDO1 and p27 expression and promoted AhR nuclear translocalization in H22 TRC tumour-bearing mice ( Supplementary Fig. 7a ). Next, we treated B16 melanoma-bearing mice with IFN-γ and an IDO1 or AhR inhibitor. As shown in Fig. 7b,c , IFN-γ and 1-MT treatment significantly decreased the percentage of cells with G0/G1 arrest from 34 to 7% and decreased TRC colony number. A similar result was obtained with IFN-γ plus DMF treatment ( Fig. 7b,c ), suggesting that blockade of the IDO-Kyn-AhR cascade plus IFN-γ indeed disrupts dormant TRCs in vivo . In our previous studies, we found that CD133 could be a marker for B16 TRCs [13] , [14] . Here, we further sorted CD133 high tumour cells from B16 melanoma, and seeded them to the soft 3D fibrin gels. We found that most cells could grow colonies. By contrast, more than 90% CD133 − B16 cells could not grow colonies in the soft 3D fibrin gels, suggesting CD133 high B16 melanoma cells belong to TRCs ( Supplementary Fig. 7b ). To verify whether IFN-γ also effects the sphere-forming capacity of these TRCs, we counted the total CD133 high tumour cells from tumour mass by flow cytometry. We found that IFN-γ neither increased the number of CD133 high melanoma cells nor promoted the colony formation of CD133 high tumour cells in the soft 3D fibrin gels, compared to PBS group ( Supplementary Fig. 7c,d ). To further investigate this mechanism of action in vivo , B16 cells isolated from the above treated mice were used for western blot analysis. Consistent with the in vitro data, the combined treatment significantly upregulated the levels of active caspases 3 and 7 ( Fig. 7d ). Moreover, the immunofluorescent staining result showed that p-STAT1 was mainly located in the cytosol of cells in the IFN-γ treated group, while the addition of 1-MT or DMF resulted in increased translocation of p-STAT1 into the nucleus ( Fig. 7e ). In addition to B16 melanoma, 1-MT and DMF treatment also disrupted IFN-γ-induced dormant H22 TRCs in the murine hepatocellular carcinoma ascites model ( Supplementary Fig. 7e,f ). Similarly, treatment with IFN-γ plus 1-MT or DMF enhanced the expression of active caspases 3 and 7 ( Supplementary Fig. 7g ), indicating that blocking IDO1-AhR pathway abrogates IFN-γ-induced dormant TRCs in vivo . In addition, three days after mice were injected with B16 TRCs, we treated these mice with IFN-γ for 20 days, and then treated the mice with DMF, 1-MT or PBS for another 20 days. From these treated groups, we found that there was no significant difference of CD133 high tumour cell number between the PBS and IFN-γ groups ( Supplementary Fig. 7h ). However, additional 1-MT or DMF treatment significantly decreased the number of CD133 high tumour cells ( Supplementary Fig. 7h ). Then, we seeded tumour cells into soft 3D fibrin gels, and found that the number of colonies in the PBS and IFN-γ groups were not different, while the colony number remarkably decreased in the 1-MT and DMF groups ( Supplementary Fig. 7i ). These results might be due to the production of endogenous IFN-γ following the 20 days of IFN-γ treatment. 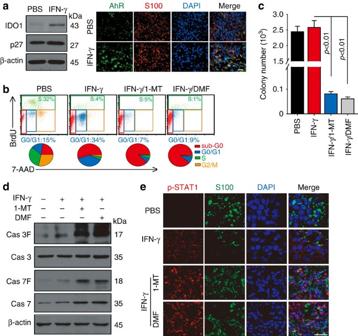Figure 7: Combining IFN-γ and an IDO or AhR inhibitor disrupts murine TRC dormancyin vivo. (a) C57BL/6 mice with 5 × 5 mm B16 melanoma were intratumorally treated with 10 μg IFN-γ once daily for 3 days (n=6 per group). Isolated primary tumour cells from a part of tumour tissue were analysed by western blot with anti-IDO1, p27 and β-actin antibody, respectively (left). Another part of tumour tissue was immunostained with anti-AhR (green), S100 (red) and DAPI (blue), and observed under confocal microscopy (right). Bar, 20 μm. (b,c) mice with 5 × 5 mm B16 melanoma were intratumorally treated with 10 μg IFN-γ, IFN-γ/1-MT (5 mg ml−1, 3–4 ml per mouse per day) or IFN-γ/DMF (10 mg kg−1) once daily for 3 days (n=6 per group). Isolated primary tumour cells were assayed for cell cycle analysis (b). The tumour cells were cultured in 3D soft fibrin gels. Four days later, the colony number was counted (c). The data represent mean±s.e.m. (analysis of Student’st-test). (d) the same asb, but isolated primary tumour cells were used to analyse caspase 3, caspase 7 and their cleaved forms by western blot (n=6 per group). (e) tumour tissue frombwere fixed in paraffin for immunocytochemical analysis with anti-p-STAT1 (red), anti-S100 (green) and DAPI (blue). Bar, 25 μm. Figure 7: Combining IFN-γ and an IDO or AhR inhibitor disrupts murine TRC dormancy in vivo . ( a ) C57BL/6 mice with 5 × 5 mm B16 melanoma were intratumorally treated with 10 μg IFN-γ once daily for 3 days ( n =6 per group). Isolated primary tumour cells from a part of tumour tissue were analysed by western blot with anti-IDO1, p27 and β-actin antibody, respectively (left). Another part of tumour tissue was immunostained with anti-AhR (green), S100 (red) and DAPI (blue), and observed under confocal microscopy (right). Bar, 20 μm. ( b , c ) mice with 5 × 5 mm B16 melanoma were intratumorally treated with 10 μg IFN-γ, IFN-γ/1-MT (5 mg ml −1 , 3–4 ml per mouse per day) or IFN-γ/DMF (10 mg kg −1 ) once daily for 3 days ( n =6 per group). Isolated primary tumour cells were assayed for cell cycle analysis ( b ). The tumour cells were cultured in 3D soft fibrin gels. Four days later, the colony number was counted ( c ). The data represent mean±s.e.m. (analysis of Student’s t -test). ( d ) the same as b , but isolated primary tumour cells were used to analyse caspase 3, caspase 7 and their cleaved forms by western blot ( n =6 per group). ( e ) tumour tissue from b were fixed in paraffin for immunocytochemical analysis with anti-p-STAT1 (red), anti-S100 (green) and DAPI (blue). Bar, 25 μm. Full size image IFN-γ plus an IDO/AhR inhibitor eliminates tumour in vivo IDO has recently been proposed to account for tumour-induced immunosuppression by oxidative cleavage of tryptophan and the generation of Kyn. As a potential cancer immunotherapeutic means, IDO inhibitors (INCB024360, GDC-0919, indoximod, and an IDO1 peptide-based vaccine) are currently in clinical trials against various types of cancers [44] . However, based on our above findings, we believe that a combination of an IDO or AhR inhibitor not only enhances antitumour immunity but also targets TRCs, leading to better treatment outcomes. In support of this idea, we found that the combination of IFN-γ and 1-MT significantly inhibited B16 melanoma tumour growth in immunodeficient NOD-SCID mice ( Fig. 8a ). In addition, when we took advantage of the endogenous IFN-γ and injected IDO1-knockdown B16 cells into wild-type mice, we found that IDO1 knockdown significantly suppressed B16 melanoma growth and prolonged the survival of mice ( Fig. 8b ), which however was effectively blunted by IFN-γ neutralizing antibody ( Fig. 8c ), further confirming that an IDO inhibitor requires the combination of IFN-γ. Then, we compared the effect of 1-MT or DMF with that of 1-MT or DMF plus IFN-γ in B16 melanoma. The melanoma-bearing mice were treated with IFN-γ plus 1-MT or DMF for 10 days. The result showed that the combined treatment was superior to each single treatment by significantly repressing tumour growth and prolonging the survival of mice ( Fig. 8d,e ). On the other hand, 1-MT showed some effect on tumour growth ( Fig. 8d ). This might be due to an inhibition of IDO which may generate an antitumour effect through an immune modulation mechanism [45] , [46] . We further dissected the tumour mass to see whether the combined treatment affects the dormancy/survival behaviour of TRCs. We found that IFN-γ treatment alone did not reduce the number of CD133 high B16 cells ( Supplementary Fig. 7d ) but resulted in most of them entering G0/G1 cell cycle arrest ( Supplementary Fig. 8a ); however, IFN-γ plus 1-MT or DMF significantly reduced CD133 high B16 cell number ( Supplementary Fig. 8b ). To further evaluate the combined therapeutic efficiency, mice with large B16 melanomas (7 × 7 mm) were treated with IFN-γ and 1-MT or DMF. In this case, the treatment efficiency was also observed with inhibited tumour growth and prolonged survival of the mice ( Supplementary Fig. 8c ). In addition to melanoma, large H22 hepatocellular carcinoma (7 × 7 mm) was also effectively treated by the combination of IFN-γ and 1-MT or DMF ( Supplementary Fig. 8d,e ), further demonstrating that IFN-γ and IDO1/AhR inhibitor have remarkable treatment efficiency. Together, these data suggest that the combination of IFN-γ and IDO1/AhR inhibitor is an ideal treatment approach against cancers, which may be independent of the adaptive immune system. 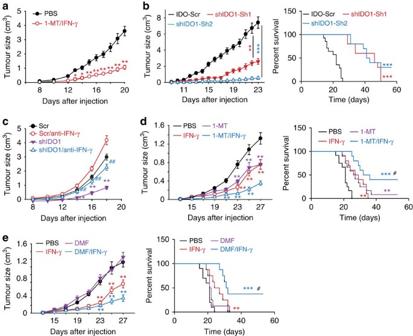Figure 8: The combining therapy of IFN-γ and 1-MT/DMF targets tumour independent of the adaptive immune system. (a) The NOD-SCID mice (n=8) with B16 melanoma (7 × 7 mm) were treated with IFN-γ/1-MT for 1 week. The tumour growth was measured. (b) IDO1-stably silencing or scramble control B16 cells (1 × 105) were s.c. injected to C57BL/6 mice (n=10 per group). The tumour growth was measured (left) and long-term survival was analysed (right). (c) IDO1-knockdown or scramble control B16 cells were injected to C57BL/6 mice (n=8 per group). Twelve hours before tumour cell injection, mice were treated with anti-IFN-γ antibody (250 μg) once every 2 days. Tumour growth was measured. (d) C57BL/6 mice (n=10 per group) were s.c. injected with 1 × 105B16 cells. Three days later, mice were treated with IFN-γ (intratumoral injection of 20 μg per day, once every 2 days), 1-MT (5 mg ml−1in drinking water, 3–4 ml per mouse per day) or IFN-γ/1-MT for 10 days. The tumour growth was measured (left) and long-term survival was analysed (right). (e) Three days after injection of 1 × 105B16 cells, C57BL/6 mice were treated with IFN-γ, DMF (intragastric injection of 10 mg kg−1, once per 2 days) or IFN-γ/DMF for 10 days (n=10 per group). The tumour growth was measured (left) and long-term survival was analysed (right). The data represent mean±s.e.m., *P<0.05, **P<0.01, ***P<0.001 versus PBS group;#P<0.05,##P<0.01 versus Scr or IFN-γ group (Student’st-test or Kaplan–Meier analysis). Figure 8: The combining therapy of IFN-γ and 1-MT/DMF targets tumour independent of the adaptive immune system. ( a ) The NOD-SCID mice ( n =8) with B16 melanoma (7 × 7 mm) were treated with IFN-γ/1-MT for 1 week. The tumour growth was measured. ( b ) IDO1-stably silencing or scramble control B16 cells (1 × 10 5 ) were s.c. injected to C57BL/6 mice ( n =10 per group). The tumour growth was measured (left) and long-term survival was analysed (right). ( c ) IDO1-knockdown or scramble control B16 cells were injected to C57BL/6 mice ( n =8 per group). Twelve hours before tumour cell injection, mice were treated with anti-IFN-γ antibody (250 μg) once every 2 days. Tumour growth was measured. ( d ) C57BL/6 mice ( n =10 per group) were s.c. injected with 1 × 10 5 B16 cells. Three days later, mice were treated with IFN-γ (intratumoral injection of 20 μg per day, once every 2 days), 1-MT (5 mg ml −1 in drinking water, 3–4 ml per mouse per day) or IFN-γ/1-MT for 10 days. The tumour growth was measured (left) and long-term survival was analysed (right). ( e ) Three days after injection of 1 × 10 5 B16 cells, C57BL/6 mice were treated with IFN-γ, DMF (intragastric injection of 10 mg kg −1 , once per 2 days) or IFN-γ/DMF for 10 days ( n =10 per group). The tumour growth was measured (left) and long-term survival was analysed (right). The data represent mean±s.e.m., * P <0.05, ** P <0.01, *** P <0.001 versus PBS group; # P <0.05, ## P <0.01 versus Scr or IFN-γ group (Student’s t -test or Kaplan–Meier analysis). Full size image Blocking IDO1-AhR abrogates dormant human TRCs by IFN-γ Next, we wondered whether the mechanism underlying IFN-γ-induced TRC dormancy was universal and could be translated to human TRCs. In this regard, a human melanoma cell line A375 was first tested. We found that consistent with the observations in B16 TRCs, human IFN-γ also induced A375 TRCs into dormancy, as evidenced by its inhibition of TRC growth, induction of cell cycle arrest at G0/G1 phase, decreased glucose consumption and absence of senescence ( Fig. 9a–d ). In addition, other human TRCs derived from MCF7 (breast cancer) and HepG2 (liver cancer) also enter dormancy driven by IFN-γ ( Supplementary Fig. 9a–d ). More importantly, primary TRCs from melanoma patient also entered dormancy by IFN-γ ( Fig. 9a–d ). To verify that IFN-γ is also inducing human TRC into dormancy through the IDO1-AhR pathway, the expression of human IDO1 was analysed by a western blot. The result showed that the expression of IDO1 was upregulated by IFN-γ in A375, MCF-7 or HepG2 control cells and further enhanced in the corresponding TRCs ( Fig. 9e and Supplementary Fig. 9e ). Meanwhile, the immunofluorescent assay showed that human IFN-γ increased both the expression and nuclear translocation of AhR in A375 and HepG2 TRCs ( Fig. 9f and Supplementary Fig. 9f ). Moreover, p27 expression was also markedly upregulated in TRCs upon IFN-γ treatment, while p-STAT1 expression was much lower in TRCs compared to control counterparts. In line with these results, the addition of kynurenine induced A375, MCF-7 and HepG2 TRCs into dormancy, which could be reversed by an AhR inhibitor ( Fig. 9g and Supplementary Fig. 9g ), suggesting that IFN-γ also induces human TRC dormancy through IDO1-AhR-p27 pathway. Significantly, combining human IFN-γ and 1-MT or DMF also abrogated dormant human TRCs, as shown by the decreased colony size and number of human TRCs ( Fig. 9h,i and Supplementary Fig. 9h,i ), which is consistent with the above findings in B16 TRCs. In support of these results, we found that IFN-γ and 1-MT had a striking treatment effect against human MCF-7 breast cancer in NOD-SCID mice ( Fig. 9j ). Together, these data suggest that IFN-γ also uses the IDO1-AhR-p27 pathway to induce human TRC dormancy. 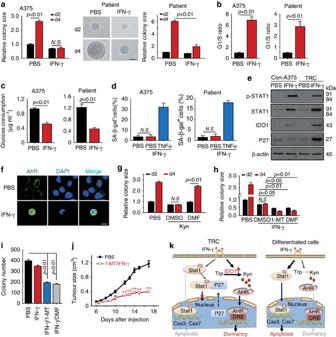Figure 9: Dormant human TRCs by IFN-γ are also abrogated by blocking IDO1-AhR pathway. (a) A375 or primary human melanoma cells were cultured in soft 3D fibrin gels for 2 days and then treated with IFN-γ (150 ng ml−1or 200 ng ml−1) for the indicated days. (b–d) A375 or primary human melanoma TRCs treated with IFN-γ for 3 days were subjected to cell cycle analysis (b), glucose consumption assay (c) or SA-β gal staining (d). (e) A375 cells grown in rigid plate or soft 3D gels were treated with IFN-γ (150 ng ml−1) for 3 days and then subjected to western blot against phospho-STAT1, STAT1, IDO1, p27 and β-actin, respectively. (f) A375 TRCs treated with IFN-γ (150 ng ml−1) were immunostained with anti-AhR antibody (green) and DAPI (blue), and observed under confocal microscope. (g) A375 TRCs were treated with Kyn (150 μM) or Kyn+DMF (20 μM) for 48 h. The colony size was calculated. (h,i) A375 cells were treated with IFN-γ (150 ng ml−1) in the presence or absence of 1-MT (0.2 mM) or DMF (20 μM) for 3 days. The colony size was quantified (h) and colony number was counted (i). (j) NOD-SCID mice (n=8 per group) with human MCF-7 breast cancer (7 × 7 mm) were treated with IFN-γ/1-MT for 1 week. The tumour growth was measured. (k) IFN-γ activates p-STAT1 pathway to trigger apoptosis in differentiated cells, while IFN-γ switches from the p-STAT1 pathway to the IDO-Kyn-AhR-p27 cascade to induce TRC dormancy. The relative colony size in this figure was calculated by comparing the colony size in other groups with the colony size in the PBS (d2) group, which was set to 1. Data shown are representative of three independent experiments and error bars represent mean±s.e.m., NS, no significant difference (Student’st-test). Figure 9: Dormant human TRCs by IFN-γ are also abrogated by blocking IDO1-AhR pathway. ( a ) A375 or primary human melanoma cells were cultured in soft 3D fibrin gels for 2 days and then treated with IFN-γ (150 ng ml −1 or 200 ng ml −1 ) for the indicated days. ( b – d ) A375 or primary human melanoma TRCs treated with IFN-γ for 3 days were subjected to cell cycle analysis ( b ), glucose consumption assay ( c ) or SA-β gal staining ( d ). ( e ) A375 cells grown in rigid plate or soft 3D gels were treated with IFN-γ (150 ng ml −1 ) for 3 days and then subjected to western blot against phospho-STAT1, STAT1, IDO1, p27 and β-actin, respectively. ( f ) A375 TRCs treated with IFN-γ (150 ng ml −1 ) were immunostained with anti-AhR antibody (green) and DAPI (blue), and observed under confocal microscope. ( g ) A375 TRCs were treated with Kyn (150 μM) or Kyn+DMF (20 μM) for 48 h. The colony size was calculated. ( h , i ) A375 cells were treated with IFN-γ (150 ng ml −1 ) in the presence or absence of 1-MT (0.2 mM) or DMF (20 μM) for 3 days. The colony size was quantified ( h ) and colony number was counted ( i ). ( j ) NOD-SCID mice ( n =8 per group) with human MCF-7 breast cancer (7 × 7 mm) were treated with IFN-γ/1-MT for 1 week. The tumour growth was measured. ( k ) IFN-γ activates p-STAT1 pathway to trigger apoptosis in differentiated cells, while IFN-γ switches from the p-STAT1 pathway to the IDO-Kyn-AhR-p27 cascade to induce TRC dormancy. The relative colony size in this figure was calculated by comparing the colony size in other groups with the colony size in the PBS (d2) group, which was set to 1. Data shown are representative of three independent experiments and error bars represent mean±s.e.m., NS, no significant difference (Student’s t -test). Full size image Despite clinically observing the immunologic dormancy of cancers in post-transplantation patients [1] , [2] , [3] , the underlying cellular and molecular mechanisms still remain unclear. Our findings demonstrate that the IDO-Kyn-AhR cascade upregulates p27 expression, leading to cell cycle arrest and TRC dormancy on one hand; the resultant p27 then binds to cytosolic p-STAT1 and might subsequently prevents its translocation into the nucleus, thus blocking IFN-γ-activated cell apoptosis on the other hand ( Fig. 9k ). In line with this molecular basis, we further provide evidence that the combination of IFN-γ and an IDO1/AhR inhibitor effectively disrupts dormant TRCs, leading to a novel tumour immunotherapeutic strategy with potential clinical applications. IFN-γ is primarily produced by CTLs and NK cells. Intriguingly, the levels of IFN-γ produced by T cells seem to be related to the effectiveness of current anti-PD-1 or CTLA4 immunotherapy in cancer patients [47] , [48] . Upon binding to the type II IFN receptor on tumour cells, IFN-γ triggers the JAK/STAT signalling cascade as well as PI3K and mTOR pathways [24] . Activation of these pathways leads to the expression of a large array of interferon-induced genes, leading to robust antitumour immune responses [49] , [50] . To date, increased levels of IFN-γ are used to explain a good outcome by upregulating the MHC class I of tumour cells, targeting endothelium and inhibiting neoangiogenesis, activating M1 macrophages and NK cells, enhancing antitumour Th1 immune response, and directly inducing tumour cell apoptosis [51] . However, our findings suggest another explanation based on IFN-γ inducing the entry of TRCs into dormancy, which might be very important, considering the tumour seed-like role of TRCs. In the present study, we elucidate the molecular basis of IFN-γ-induced TRC dormancy, which involves IDO-Kyn-AhR cascade. Nevertheless, this molecular pathway might reflect the interaction between cells and their environment during evolution. Ancestral cells face two major forms of danger, biological pathogens and non-biological chemical toxins. Undoubtedly, either clearance of the invader or killing the cell may be the consequence. However, for certain pathogens or xenobiotic substances, cells neither clear them quickly nor are killed by them. Cells thus might develop a strategy to counteract sub-toxic invaders by entering dormancy and waking up after spontaneous clearance of the invaders. Since cells evolved the interferon pathway to defend pathogens, and use AhR as an arm against chemical toxins [52] , [53] , it is possible for ancestral cells to evolve using IFN-IDO-Kyn-AhR as a common means to trigger cellular dormancy against those subtoxic pathogenic and xenobiotic invaders. On the other hand, it is reasonable to speculate that TRCs as stem cell-like cells might possess some similarity to ancestral cells, thus inheriting IDO-Kyn-AhR cascade. In fact, both IDO1 and AhR are very conserved molecules [54] , [55] . Recently, the concept that immune cells can endow stem-like properties of tumour cells have been substantiated by both human Th22 and MDSCs that can induce cancer stemness via distinct molecular mechanisms in human colon and ovarian cancer, respectively [56] , [57] . Nonetheless, the present study indicates that effector T cells and NK cells may also induce tumour stemness via IFN-γ-mediated TRC dormancy, which thus extends previous studies to antitumour effector immune cells. A key issue about tumour cell dormancy is whether it is only associated with TRCs rather than with differentiated tumour cells, which is supported by recent studies [17] , [58] . Our current study further supports this idea by confirming that IFN-γ has a differential effect on differentiated tumour cells and TRCs, inducing the former to enter apoptosis but the latter to enter dormancy. Intriguingly, this IFN-γ-induced TRC dormancy seemingly could be shifted to senescence in concert with TNF-α signalling [59] . Although IFN-γ-induced TRC dormancy is mediated by the IDO-Kyn-AhR cascade, this process actually requires enough tryptophan supplement to generate Kyn. Tryptophan is an essential amino acid that cannot be synthesized by cells. Intriguingly, in another study we found that IFN-γ-treated TRCs did not decrease intracellular levels of tryptophan due to increased uptake of tryptophan via upregulating its transporter, which was, however, downregulated in differentiated tumour cells. Accordingly, the present study revealed high and low levels of IDO1 and AhR in TRCs and differentiated tumour cells, respectively, regardless of IFN-γ stimulation. Thus, the differential expression pattern of tryptophan, IDO1 and AhR may explain why IFN-γ induces TRCs rather than differentiated tumour cells to enter dormancy. In fact, in line with this expression pattern, we found that in response to IFN-γ stimulation, differentiated tumour cells were biased towards the JAK-STAT1 pathway, while TRCs preferred to activate the IDO-Kyn-AhR cascade ( Fig. 9k ). Such a difference might be due to a pre-existing potential activity to metabolize tryptophan in TRCs. Compared to differentiated tumour cells, TRCs expressed much higher IDO1 and AhR ( Fig. 5a,b and Supplementary Fig. 3a ). In addition, in another study, we also found that compared to differentiated tumour cells, TRCs expressed much higher levels of a tryptophan transporter on their membrane surface that transports tryptophan into the cytosol of TRCs. Although IFN-γ can upregulate the expression of IDO1 in differentiated tumour cells, due to the relatively low levels of IDO1, tryptophan transporter and AhR, there is not enough Kyn to activate AhR. In contrast, when IFN-γ stimulates TRCs, the phosphorylated STAT1 can rapidly upregulate the expression of both IDO1 and AhR, leading to the production of high levels of Kyn and the subsequent activation of AhR. Interestingly, a recent study showed that the activation of Kyn-AhR signalling pathway only requires IFN-γ at the beginning [60] . An important finding from this study is that although activation of the IDO-Kyn-AhR cascade by IFN-γ leads to TRCs entering dormancy and escaping immunosurveillance, switching the IDO-Kyn-AhR cascade to JAK-STAT1 signalling may result in disruption of dormant TRCs. Activation of the IDO-Kyn-AhR cascade upregulates the expression of p27, a key cell cycle inhibitor. Intriguingly, we found that p27 may directly bind phosphorylated STAT1, thus making TRCs biased towards the IDO-AhR cascade. By contrast, blockade of p27 may switch the IDO-Kyn-AhR cascade to the JAK-STAT1 pathway, a signalling that may induce apoptosis via caspases 2, 3 and 7 (refs 42 , 43 ). Indeed, we observed the activation of caspases 3 and 7 by IFN-γ in this present study. Meanwhile, either IDO1 or AhR inhibitor overtly induced IFN-γ-mediated translocation of STAT-1 into the nucleus of TRCs. We thus combined IFN-γ and IDO1 or AhR inhibitor to switch IDO-Kyn-AhR cascade to STAT1 signalling to target dormant TRCs. Therapeutically, ideal outcomes were achieved in different tumour models, including in immunodeficient NOD-SCID mice, which further support that combining IFN-γ and an IDO1 or AhR inhibitor directly target dormant TRCs. Although this mechanism elucidation provides us deep understanding of the role of IFN-γ in tumour, its concentration actually is another critical issue. In an in vitro experiment, we found that only a high concentration (>50 ng ml −1 ) of IFN-γ is capable of inducing TRC dormancy. In general, physiological IFN-γ probably cannot reach such high concentration in vivo . However, during the direct interaction of effector T or NK cells with TRCs, a high concentration of IFN-γ might be formed at the local immune synapse site, leading to TRC dormancy. The generation of high levels of IFN-γ at the local synapse site might be regulated by the stages of tumour. Since tumours at their early stage generate much less immunosuppressive factors, effector T or NK cells could be optimally activated and produce a large amount of IFN-γ. By contrast, tumours at their late stage generate much more immunosuppressive factors, which impede the production of IFN-γ by T or NK cells. However, low levels of IFN-γ can stimulate immune cells such as macrophages and DCs to upregulate the expression of IDO1 and PD-L1 to mediate immunosuppression [61] , [62] . Identification of such a combined therapy of IFN-γ and an IDO1 or AhR inhibitor may be very significant for current cancer immunotherapy. In clinical practice, neither adoptive T-cell therapy nor check point blockade therapy or oncolytic virotherapy are efficient to attack TRCs. Thus, TRCs’ immune evasion may lead to treatment failure regarding their roles in tumour recurrence, metastasis and drug resistance. In fact, tumour recurrence was reported after PD-1 antibody treatment in certain melanoma and lung cancer patients, which might be explained by TRCs escaping immunotherapy [63] , [64] . Notably, a recent review by Zou et al . emphasized the link of clinical PD-L1/PD-1 blockade resistance to potential cancer dormancy (stemness), further suggesting the significance of targeting TRC dormancy in tumour immunotherapy [65] . On the other hand, clinical disease-free cancer patients after treatment might be interpreted as IFN-γ inducing TRC dormancy. In this study, we found that when TRC dormancy was triggered by high dose IFN-γ, such dormancy could be maintained by low-dose IFN-γ. In our another study on tumour vaccine, although no tumour formed at the tumour inoculation site, low levels of IFN-γ were found to be continually expressed there. Thus, it is necessary to clarify whether the disease-free status is mediated by IFN-γ in those cancer patients. On the other hand, IDO-targeting interventions have already entered clinical trials in cancer patients [66] , and their antineoplastic effects were taken for granted due to their reactivating antitumour immunosurveillance. However, our present findings suggest that the clinically observed antitumour effects might be largely due to targeting dormant TRCs by blocking the IDO-AhR cascade in the presence of endogenous IFN-γ. It will be interesting to compare IFN-γ levels in IDO1 inhibitor-responsive cancer patients with that in unresponsive ones. For this combined treatment, an important issue is how to efficiently deliver IFN-γ and IDO or DMF inhibitor to the tumour site. In this study, we found that although IFN-γ/IDO or DMF inhibitor effectively treated tumours, they still grew. This might be due to the unequal distribution of IFN-γ and IDO or DMF inhibitor in the tumour mass, leading to part of the TRCs left behind. Alternatively, certain heterogenous TRCs are likely not sensitive to the effects of the IFN-γ signalling pathway. In summary, the data in this study clearly show that IFN-γ, by virtue of its activating the IDO-Kyn-AhR cascade, induces dormancy in TRCs, leading to the discovery of the combination of IFN-γ and an IDO1 or AhR inhibitor effectively attacking dormant TRCs. This study may open a new venue for cancer immunotherapy. Animals and cell lines Female C57BL/6, BALB/c mice and NOD-SCID mice, 6–8 weeks old, were purchased from Center of Medical Experimental Animals of Chinese Academy of Medical Science (Beijing, China). OT-I transgenic mice were gifted by Dr Hui Zhang (Sun Yat-Sen University). These animals were maintained in the Animal Facilities of Chinese Academy of Medical Science under pathogen-free conditions. All studies involving mice were approved by the Animal Care and Use Committee of Chinese Academy of Medical Science. Mouse tumour cell lines B16 (melanoma), OVA-B16 (melanoma), CT26 (colon cancer) and H22 (hepatocellular carcinoma), and human tumour cell lines A375 (melanoma), MCF-7 (breast cancer), HepG2 (liver cancer) and HEK-293T (human embryonic kidney) were purchased from China Center for Type Culture Collectin (Beijing, China) and cultured in DMEM (Thermo Scientific) with 10% fetal bovine serum (FBS) (Gibco, USA), except that H22 cells were grown in RPMI1640 medium (Gibco, USA) with 10% FBS. Cells were tested for mycoplasma detection, inter-species cross contamination and authenticated by isoenzyme and short tandem repeat (STR) analyses in Cell Resource Centre of Peking Union Medical College before the beginning of the study and spontaneously during the research. 2D rigid dish and 3D fibrin gel cell culture of tumour cells For conventional 2D cell culture, tumour cells were maintained in rigid dish with MEM cell culture medium supplemented with 10% FBS (Invitrogen, Carlsbad, CA, USA) at 37 °C with 5% CO 2 . TRC culture was conducted according to our previously described method (Liu et al ., 2012). In brief, tumour cells were maintained in the conventional rigid plate. After 0.25% trypsin digestion, cells were detached and suspended in DMEM (10% FBS) and cell density was adjusted to 10 4 cells ml −1 . Fibrinogen (Searun Holdings Company, Freeport, ME, USA) was diluted into 2 mg ml −1 with T7 buffer (pH 7.4, 50 mM Tris, 150 mM NaCl). A 1:1 fibrinogen and cell solution mixture was made by mixing the same volume of the fibrinogen solution and the cell solution, resulting in 1 mg ml −1 fibrinogen and 5,000 cells ml −1 in the mixture. 250 μl cell per fibrinogen mixtures was seeded into each well of 24-well plate and mixed well with pre-added 5 μl thrombin (0.1 U μl −1 , Searun Holdings Company). The cell culture plate was then moved into 37 °C cell culture incubator and incubated for 30 min. Finally, 1 ml DMEM medium containing 10% FBS and antibiotics were added. On day 5, the cells cultured in soft 3D fibrin gels (90 Pascal) were treated with dispase II (Roche, Swiss) for 10 min at 37 °C and then the spheroids were collected and pipetted to single cells. Plasmids and reagents pGFP-C-shLenti-shIDO1, pLenti-C-Myc-DDK-IDO1, pGFP-C-shLenti-shAHR, pCMV6-AHR and pGFP-C-shLenti-shSTAT1 were purchased from Origene (MD, USA). pX330-p27SGRNA and pX330-GCN2SGRNA plasmids were purchased from Addgene (MA, USA). Kynurenine, 1-L-MT, methotrexate (MTX), paclitaxel (PAX), kynurenic acid, indoxyle sulphate, melatonin, aspartame and DMF were from Sigma-Aldrich (ST, USA). IFN-γ and anti-IFN-γ neutralized antibody were purchased from PeproTech (Rocky Hill, NJ, USA). Salmon fibrinogen, thrombin and dispase were from Reagent Proteins (CA, USA). Fludarabine was from Selleck Company (Shanghai, China). Puromycin was from Invitrogen (SD, USA). Generation of OVA-specific CD8 + T cells Ovalbumin (OVA)-specific CD8 + T cells were isolated from the spleen of OT-I transgenic mice by positive selection using magnetic cell separation (MACS, mouse naïve CD8 + T-cell Isolation Kit, Miltenyi Biotec). Above 95% purity was confirmed by flow cytometry using anti-CD8 antibody (eBioscience, CA, USA). The isolated CD8 + T cells were cultured in RPMI 1640 medium containing 10% FBS and 100 U ml −1 IL-2 (eBioscience, CA, USA) and activated by the addition of anti-CD3 and anti-CD28 (1 μg ml −1 each). Cytokines release and Kyn production Cytokine production in the supernatants was quantified by ELISA kits (eBiosence, CA, USA) according to the manufacturer’s protocol and Kyn production was measured by ELISA (MYBioSource, CA, USA) according to the supplier’s instructions. Transient and stable transfection of shRNAs Transient transfection of B16 TRCs was performed with RNAimax reagent (Invitrogen) following the manufacturer’s instructions. Stable IDO1-shRNA, AhR-shRNA or STAT1-shRNA cell lines were generated by lentiviral transduction and selected by flow cytometry sorting. Briefly, Pspax2, pVSV-G and pGFP-C-shLenti-shIDO1, pGFP-C-shLenti-shAhR, pGFP-C-shLenti-shSTAT1 or scrambled control were transfected into HEK 293T cells using FuGENE HD transfection reagent (Roche). The supernatants containing viruses were mixed with polybrene to a final concentration of 8 μg ml −1 before infection of B16 cells. Cells with stable knockdown of IDO1, AhR or STAT1 were sorted with FACS and cultured in 0.5 μg ml −1 puromycin with 10% FBS. The following shRNAs from Origene were used: scrambled shRNA: 5′-GCACTACCAGAGCTAACTCAG ATAGTACT-3′ (sense) and 5′-AGTACTATCTGAGTTAGCTCTGGTAG TGC-3′ (antisense); IDO1 shRNA1, 5′-TCCTAAGGAGTGTGAAAGATACAACCGAG-3′ (sense) and 5′-CTCGGT TGTATCTTTCACACTCCTTAGGA-3′ (antisense); IDO1 shRNA2, 5′-AAACACGAGGCT GGCAAAGAATCTCCTGC-3′ (sense) and 5′-GCAGGAGATTCTTTGCCAGCCTCGTG TTT-3′ (antisense); AhR shRNA1, 5′-CCAACATCACCTATGCCAGCCGCAAGCGG-3′ (sense) and 5′-CCGCTTGCGGCTGGCATAGGTGATGTTGG-3′ (antisense); AhR shRNA2, 5′-GGTT CTCAGGCATTCCTAAGCAAGGTGCA-3′ (sense) and 5′-TGCACCTTGCTTAGGAATGCCTGAGAACC-3′ (antisense); STAT1 shRNA1, 5′-CTCCTTCGTGGTAGAACGACAGC CGTGCA-3′ (sense) and 5′-TGCAC GGCTGTCGTTCTACCACGAAGGAG-3′ (antisense); STAT1 shRNA2, 5′-AAGAATCCACCAACGGAAGTCTGGCAGCT-3′ (sense) and 5′-AGCTGCCAGACTTCC GTTGGTGGATTCTT-3′ (antisense). For construction of the stable knockdown of p27-B16 or GCN2-B16 cell line, B16 cells were transfected with Linear Selection Markers-puromycin resistance (Clontech, CA, USA) and pX330-U6-Chimeric_BB-CBh-hSpCas9-p27-SGRNA1, pX330-U6-Chimeric_BB-CBh-hSpCas9-p27-SGRNA2, pX330-U6-Chimeric_BB-CBh-hSpCas9-GCN2-SGRNA1, or pX330-U6-Chimeric_BB-CBh-hSpCas9-GCN2-SGRNA2 (Addgene, MA, USA) for 24 h. The following primers were used: SGGFP: 5′-CACCGGGGCGAGGAGCTGTTCACCG-3′ (sense) and 5′-AAACCGGTGAACAGCTCCTCGCCCC-3′ (antisense); p27-SGRNA1, 5′-CACCGGCGGATGGACGCCAGACAAG-3′ (sense) and 5′-AAACCTTGTCTGGCGTCCATCCGCC-3′ (antisense); p27-SGRNA2, 5′-CACCGTGG GTCTCAGGCAAACTCTG-3′ (sense) and 5′-AAACCAGAGTTTGCCTGAGACCCAC-3′ (antisense); GCN2-SGRNA1, 5′-CACCGGCT CGGACTTCCAGGATCTG-3′ (sense) and 5′-AAACCAGATCCTGGAAGTCCGAGCC-3′ (antisense); GCN2-SGRNA2, 5′-CACCGCGCTGCGAATAGCTCTCCTG-3′ (sense) and 5′-AAACCAGGAGAGCTATTCGCAGCGC-3′ (antisense). Cells were then selected with puromycin (1 μg ml −1 ) for 2 weeks and maintained in puromycin (0.5 μg ml −1 ). For constructing stable overexpression cells, B16 cells were transfected with pLenti-C-Myc-DDK-IDO1 or empty vector by using FuGENE HD transfection reagent (Roche). Cellular populations expressing Myc-IDO1 or Myc-vector were sorted by FACS and cultured with 0.5 μg ml −1 puromycin. RT–PCR Total RNA was extracted from cells using Trizol (Invitrogen) and was transcribed to cDNA by using a high capacity cDNA reverse transcription kit (Applied Biosystems, CA, USA). The primer sequences are shown as follows: IDO1, 5′-GAGGATGCGTGACTTTG TGG-3′ (sense) and 5′-ATCAAGACTCTGGAAGATGCTG-3′ (antisense); PCNA, 5′-GTCTCCTT GGTACAGCTTACTC-3′ (sense) and 5′-GTGTCTGCATTATCTTCAGCC-3′ (antisense); PD-L1, 5′-AGTATGGCAGCAACGTCACG-3′ (sense) and 5′-TCCTTTTCCCAGTACACCACTA-3′ (antisense); iNOS, 5′-GTTCTCAGCCCAACAATACAAGA-3′ (sense) and 5′-GTGGACGGGT CGATGTCAC-3′ (antisense); p27, 5′-TCAAACGTGAGAGTGTCTAACG-3′ (sense) and 5′-CC GGGCCGAAGAGATTTCTG-3′ (antisense); GAPDH, 5′-AGGTCGGTGTGAACGGATTTG-3′ (sense) and 5′-TGTAGACCATGTAGTTGAGGTCA-3′ (antisense). Real-time PCR was performed using ABI stepone plus (Applied Biosystems, MA, USA). Values are means±s.e.m. from three independent experiments which were performed in duplicate. Statistical comparisons among groups were performed using ANOVA followed by Fisher’s PLSD. Values of all parameters were considered statistically significant difference at a value of P <0.05. Western blotting Cells were collected, lysed in M2 lysis buffer and sonicated and protein concentrations were determined by the BCA kit (Applygen Technologies Inc., China). Then, the protein was run on an SDS–PAGE gel and transferred to nitrocellulose. Nitrocellulose membranes were blocked in 5% bovine serum albumin (BSA) and probed with antibodies overnight: anti-actin (Cell Signaling, Cat No. 3700; 1:1,000) and TopBP1 (Sigma, PLA0030, 1:1,000, ST, USA); anti-caspase 3 (Cell Signaling, Cat No. 9662; 1:1,000), cleaved caspase 3 (Cell Signaling, Cat No. 9664; 1:1,000), caspase 7 (Cell Signaling, Cat No. 9492; 1:1,000), cleaved caspase 7 (Cell Signaling, Cat No. 9491; 1:1,000), p27 (Cell Signaling, Cat No. 3686; 1:2,000), phospho-STAT1(Cell Signaling, Cat No. 9167; 1:1,000) and STAT1 (Cell Signaling, Cat No. 9172; 1:1,000); anti-β3 tubulin (Millipore, ab9354; 1:2,000, MA, USA) and IDO1 (Millipore, MABF850; 1:1,000, MA, USA) and anti-AhR abcam, ab2769, 1:1,000) and GCN2 (Abcam, ab137543; 1:1,000). Secondary antibodies conjugated to horseradish peroxidase were followed by enhanced chemiluminescence (Thermo fisher, 1:5,000, MA, USA). Results were confirmed by at least three independent experiments. Luciferase assays Hepa1-6 cell line, stably integrated with pGL3-CYP1A1 promoter-driven luciferase, were treated with different doses of Kyn for 24 h. Then, these cells were lysated and analysed by a luciferase assay using the luciferase assay kit (Promega, WI, USA) on a GloMax Multi Plus (Promega). B16 cells were transfected with 100 ng Renilla luciferase, 1 μg firefly luciferase plasmid pGL3-p27 promoter-luc and 1 μg of either vector or pCMV6-AhR for 12 h. Then, these cells were treated with or without Kyn (150 μM) for 24 h. Cells lysates were analysed using the Dual Luciferase Reporter Assay (Promega) on a GloMax Multi Plus (Promega). Firefly luciferase activity was normalized to Renilla luciferase. SA-β-gal activity assay B16 TRCs were fixed for 15 min at room temperature, and then stained overnight at 37 °C using the β-Galactosidase Staining Kit (CST, MA, USA). SA-β-gal-positive and negative cells were then counted under the microscope. Cell cycle analysis Cells were incubated with 50 μM BrdU (BD Bioscience) for 1 h and cell cycle analysis was performed using BD Pharmingen APC-BrdU Flow Kits according to the manufacturer’s protocol (BD Bioscience, NJ, USA). The samples were analysed by flow cytometry on a BD Accuri C6 Flow Cytometer (BD Bioscience). The following cell cycle phases were determined as a percentage of the total population: sub-G0 (apoptotic cells), G0/G1 (2n, BrdU-negative), S (2n to 4n, BrdU-positive) and G2/M phase (4n, BrdU-negative). In some experiments, BrdU (1 mg, BD Bioscience, NJ, USA) was i.p. injected into mice 18 h before mice were killed. The primary tumour cells were isolated from tumour or ascites and used for cell cycle analysis. Cell fractionation Cells were collected and washed twice in cold PBS. Then, the cytoplasmic and nuclear protein were isolated by using the Cell Fractionation kit (BioVison, SF, USA) according to the supplier’s instruction [67] . Equal cell equivalents were run on SDS–PAGE gels and immunoblotted. Immunofluorescence Cells were plated on fibronectin (1 μg ml −1 )-coated coverslips, fixed in 4% paraformaldehyde and permeabilized with 0.2% Triton X-100. Fixed cells were blocked in 5% BSA and probed with monoclonal anti-AhR, phospho-STAT1, Ki 67, (Abcam, UK), or anti-CD133 (eBioscience) antibody in 5% BSA, followed by Alexa Fluor 488-conjugated chicken anti-mouse (Invitrogen, CA, USA). Cells were mounted with Vectashield mounting media containing DAPI (Vector Laboratories, CA, USA). Confocal microscopy was performed on a Leica laser scanning confocal microscope. CD133 + tumour cells sorting The fresh tumour tissue removed from mice was digested with collagenase and hyaluronidase for 1 h. After grinding with semi-frosted slides and lysis of RBC, the dissociated cells were spun down at 500 r.p.m. for 1 min and then incubated for 1 h to get rid of adhesive cells. The suspended cells were stained with PE conjugated anti-CD133 antibody at room temperature for 30 min. After washing, these cells were filtered through a 40 μm cell strainer (JET Biofil, China) to obtain single cell suspension for sorting on a BD FACSARIA III (BD Bioscience, NJ, USA). Animal experiments and treatment protocol Female C57BL/6, BALB/c or NOD-SCID mice (6–8 weeks) were injected s.c. with 1 × 10 5 B16 cells, 2 × 10 5 H22 cells, 5 × 10 3 B16 TRCs, 1 × 10 5 shIDO1-Sh1-B16 cells or 1 × 10 5 shIDO1-Sh2-B16 cells into the right flank. Three days later after inoculation or after tumour growth up to 5 × 5 mm or 7 × 7 mm, mice were randomized into different groups (sample size was n =5–10) based on similar tumour size and body weight. And then, these mice were treated with or without CD8 + T cells (1 × 10 7 cells, twice), IFN-γ (intratumoral injection of 10–20 μg per day, once every 2 days), 1-MT (5 mg ml −1 in drinking water, 3–4 ml per mouse per day), IFN-γ/1-MT, DMF (intragastric injection of 10 mg kg −1 , once every 2 days), IFN-γ/DMF or anti-IFN-γ neutralizing antibody (250 μg per mouse) for the indicated time. The mice of control groups received an equal volume of saline. The incidence of tumour in mice and the survival of mice was recorded. In some experiments, mice were killed and tumours were dissected and weighed or fixed in 37% formalin on the indicated day after inoculation. In some experiments, female BALB/c mice (6–8 weeks) were inoculated with H22 cells by intraperitoneal injection and treated with or without IFN-γ (20 μg per day) for 3 days. Tumour volume was calculated according to the formula: tumour volume=length × width 2 /2. No blinding was performed. Histological and immunohistochemical staining The subcutaneous tissues of inoculation sites in mice were surgically excised, fixed in 37% formalin, embedded in paraffin and sectioned for H&E staining. Immunohistochemistry was performed by using the Vectastain Universal Elite ABC kit (Vector Laboratories, CA, USA) according to the supplied instructions. The sections from paraffin embedded tissues were incubated with anti-S100 β (1:200, Millipore, MA, USA) at 4 °C overnight. After development, tissue sections were moderately counterstained with methyl green. In some experiments, immunohistochemistry was implemented by using Tyramide Signal Amplification Plus Cyanine 3/Fluorecein system (PerkinElmer, CA, USA) according to the supplier's instructions. In brief, the sections were dewaxed, rehydrated, quenched endogenous peroxidase, blocked and incubated with anti-S100 β (1:3,000, Millipore, MA, USA), anti-AhR (1:3,000, Abcam, UK), anti-CD133 (Invitrogen, CA, USA), anti-Ki67 (Abcam, UK) and anti-p-STAT1 (1:3,000, CST, MA) at 4 °C overnight. Slides were then incubated sequentially with two HRP-conjugated secondary antibodies for 1 h at room temperature. After developing in Tyramide Signal Amplification Plus Working Solution for 5 min, the slides were counterstained with DAPI and mounted for confocal analysis. Isolating primary human melanoma cells Melanoma tissues were taken from patients. The study was approved by the Clinical Trial Ethics Committee of Peking Union Medical College. All patients have provided written informed consent to participate in the study. These tissues were cut into small pieces of 1–3 mm and minced in RPMI 1640 medium supplemented with collagenase (Sigma, 32 μg ml −1 ), hyaluronidase (Sigma, 500 μg ml −1 ) and DNAase I (Sigma, 5 μg ml −1 ). These samples were incubated for 1 h at 37 °C under continuous rotation. After digestion, the samples were filtered through Cell Strainer (BIOFIL). After centrifuged and lysized in RBC lysis buffer, the tumour cells were resuspended in RPMI1640 medium with 10% FBS, penicillin and streptomycin. The primary melanoma cells were confirmed by immunostaining with anti-S100 β antibody. Statistics analysis All experiments were performed at least three times. To determine the colony size, at least 20 colonies from different field were measured. Results are expressed as mean±s.e.m. and analysed by Student’s t -test. The P value<0.05 was considered statistically significant. The analysis was conducted using the Graphpad 6.0 software. Sample exclusion was never carried out. Data availability The authors declare that all the data supporting the findings of this study are available within the article and its Supplementary Information files and from the corresponding author on reasonable request. How to cite this article: Liu, Y. et al . Blockade of IDO-kynurenine-AhR metabolic circuitry abrogates IFN-γ-induced immunologic dormancy of tumor-repopulating cells. Nat. Commun. 8 , 15207 doi: 10.1038/ncomms15207 (2017). Publisher’s note : Springer Nature remains neutral with regard to jurisdictional claims in published maps and institutional affiliations.